The long-chain alkane metabolism network ofAlcanivorax dieselolei Alkane-degrading bacteria are ubiquitous in marine environments, but little is known about how alkane degradation is regulated. Here we investigate alkane sensing, chemotaxis, signal transduction, uptake and pathway regulation in Alcanivorax dieselolei . The outer membrane protein OmpS detects the presence of alkanes and triggers the expression of an alkane chemotaxis complex. The coupling protein CheW2 of the chemotaxis complex, which is induced only by long-chain (LC) alkanes, sends signals to trigger the expression of Cyo, which participates in modulating the expression of the negative regulator protein AlmR. This change in turn leads to the expression of ompT1 and almA , which drive the selective uptake and hydroxylation of LC alkanes, respectively. AlmA is confirmed as a hydroxylase of LC alkanes. Additional factors responsible for the metabolism of medium-chain-length alkanes are also identified, including CheW1, OmpT1 and OmpT2. These results provide new insights into alkane metabolism pathways from alkane sensing to degradation. Hydrocarbon-degrading bacteria are ubiquitous in marine environments. Some bacterial species are highly specialized to degrade hydrocarbons and are called hydrocarbonoclastic bacteria [1] , such as Alcanivorax [2] , Thalassolituus [3] , Oleiphilus [4] and Oleispira [5] . They have evolved mechanisms adapted to various marine environments, such as the cold adaptation of Oleispira antarctica [6] and the stress responses (ultraviolet irradiation), osmoregulation and nutrient scavenging of Alcanivorax borkumensis [2] , [7] , and they play a major role in marine oil pollutant removal [1] , [8] , [9] , [10] . In the past decade, studies addressing the mechanisms underlying bacterial alkane degradation have primarily focused on the enzymes involved in the initial step of oxidizing n -alkanes, particularly alkanes with short- and medium-length chains [11] , [12] , [13] , [14] . The degradation mechanisms associated with long-chain (LC) and branched alkanes are less well understood. The bacterial sensing, signal transduction, chemotaxis and absorption mechanisms involved and how alkane degradation is regulated remain virtually unknown for all alkanes [15] . Alcanivorax species are the most important alkane-degrading bacteria in marine environments [6] , [7] , [8] . In addition to A. borkumensis , A. dieselolei is another intensively studied bacterium in this genus. A. dieselolei bacteria can be found in both coastal and pelagic sea regions, from the sea surface to varying depths, and from tropical to polar areas [16] , [17] , [18] , [19] , [20] . As the type strain of A. dieselolei (MCCC 1A00001 T =DSM 16502 T ), strain B5 actively degrades numerous alkanes (C 6 –C 36 ), including branched alkanes [21] , [22] . It produces a novel lipopeptide as a biosurfactant that accelerates oil uptake [23] . This strain encodes a complex alkane monooxygenase system that includes three membrane-bound non-haeme iron alkane hydroxylases (AlkB), one cytochrome P450 (CYP) and a putative flavin-binding monooxygenase (AlmA) [22] . AlmA is postulated to be responsible for LC alkane degradation [16] . Although multiple alkane utilization pathways can coexist in a single bacterium, how they are coordinated is unclear. Several transcriptional activators have been identified in Acinetobacter, Alcanivorax and Pseudomonas species. These activators are typically encoded by alkane monooxygenase gene clusters [13] , [24] , [25] , [26] , [27] , but their regulation has rarely been investigated. In Pseudomonas aeruginosa , two alk genes are differentially expressed in response to C 10 –C 22 n -alkanes [26] , but the mechanism underlying this differential expression is unknown. In P. putida , AlkB genes may be controlled by the global regulatory protein Crc [28] . However, the crc gene is absent from the genomes of A. dieselolei B5 (CP003466) [29] and A. borkumensis SK2 (AM286690) [2] . The mechanisms that control the early responses of bacterial cells to alkanes, such as alkane sensing, chemotaxis and uptake, remain to be elucidated. Although alkane chemotaxis has been observed in bacterial isolates of Flavimonas oryzihabitans [30] and P. aeruginosa PAO1 (ref. 31 ), the underlying machinery has not been identified [32] . In addition, alkane uptake is an essential step before utilization, but the mechanism by which uptake occurs is also unknown. It has been proposed that the direct uptake of soluble alkanes is facilitated by surfactants [13] . For aromatic hydrocarbons, certain factors that enable transport across the outer membrane have been identified [33] , [34] , [35] , [36] . Apart from the terminal oxidation pathway initiated by AlkB and P450 alkane hydroxylase, the majority of the network remains undetermined, including alkane sensing, chemotaxis, differential regulation and cross-membrane transport. To understand the early responses that occur in the presence of alkanes, we have created a random genome mutation library of A. dieselolei B5. Using the mutation library, we screened and identified genes in bacterial mutants with abnormal growth in the presence of different alkanes. We further determined the roles of the mutated genes in alkane sensing, chemotaxis and uptake, and the regulation and coordination of different alkane utilization pathways. Genes involved in utilizing LC alkanes in the B5 strain Using a high-throughput screening method, 17 mutant strains were identified from the transposon mutant library that exhibited abnormal (absent or increased) growth with C 32 as the sole carbon source but wild-type-like growth with acetate as the sole carbon source. 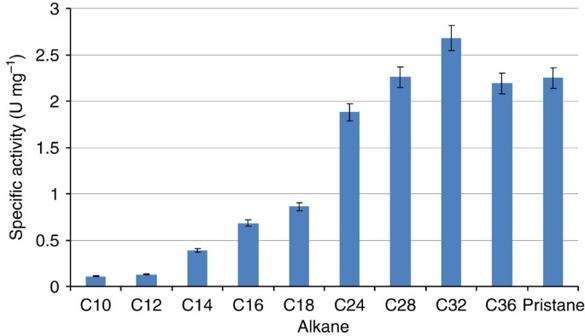Figure 1: Enzymatic activity of LC-alkane monooxygenase AlmA showing the substrate range of alkanes with different chain lengths. The purified AlmA was assayed for alkane monooxygenase activity using the method described in the Methods section. Enzymatic activity is expressed as U mg−1enzyme. One unit was defined as the amount of enzyme required for hydroxylation of 1 μmol of alkane per min. The values presented are the averages of three independent experiments. Error bars represent the s.d. The transposon insertion sites and corresponding interrupted genes (13 in total) were identified in these mutants ( Table 1 ). The disrupted genes encoded one putative monooxygenase, two proteins involved in regulation, two proteins involved in secretion, three proteins involved in chemotaxis, three proteins responsible for LC fatty acid transportation and two proteins with unknown function. A BLAST search in GenBank revealed that most of the genes had homologues in other Alcanivorax strains, such as in A. borkumensis SK2, for which the full genome has been sequenced [2] . Complementation experiment results confirmed that the LC alkane degradation deficiencies of the above mutants were not caused by a polar effect on the genes downstream of the corresponding interrupted genes ( Supplementary Fig. 1 ). Table 1 Genes identified as responsible for alkane degradation in the A. dieselolei B5 transposon mutant library. Full size table AlmA, a monooxygenase that hydroxylates alkanes In a mutant strain (MAB5) that is unable to utilize LC alkanes, we identified a transposon insertion in the almA gene ( orf B5T_02052). The almA gene has been annotated as encoding a monooxygenase ( Table 1 ). Three open reading frames flanking almA have been annotated as a hydrolase, a hypothetical regulator protein and a LC fatty acid transporter. This gene cluster is illustrated in Supplementary Fig. 2a . To verify the function of almA in alkane utilization, the growth of the almA mutant strain MAB5 was assayed using various alkanes as the sole carbon source based on the observation of the cell culture density. The results indicated that the mutant strain did not grow on C 32 or C 36 n -alkanes; grew poorly on C 24 , C 28 and pristane alkanes (C 19 H 40 ); and grew normally on C 8 , C 12 and C 16 alkanes ( Supplementary Fig. 3 ). These findings suggested that AlmA was responsible for the utilization of LC and branched alkanes in the B5 strain. To further verify the function of the almA gene, it was expressed heterologously. The purified AlmA protein was then subjected to an enzyme activity assay using various alkanes. The method applied to assay alkane monooxygenase activity is described in the Methods section. The obtained alkane transformation products revealed that the purified AlmA protein converted C 14 –C 36 alkanes and pristane to their corresponding primary alcohols ( Fig. 1 and Supplementary Fig. 4 ), as determined via gas chromatography (GC) and GC-mass spectrometry (MS). A high-specific activity was observed on C 24 –C 36 and pristane alkanes, and minimal specific activity was observed on C 10 , C 12 and C 14 alkanes. Figure 1: Enzymatic activity of LC-alkane monooxygenase AlmA showing the substrate range of alkanes with different chain lengths. The purified AlmA was assayed for alkane monooxygenase activity using the method described in the Methods section. Enzymatic activity is expressed as U mg −1 enzyme. One unit was defined as the amount of enzyme required for hydroxylation of 1 μmol of alkane per min. The values presented are the averages of three independent experiments. Error bars represent the s.d. Full size image AlmR, a gene regulatory protein of LC-alkane metabolism In a mutant library screen, the mutant strain MRB5 exhibited better growth than the wild-type strain when a C 32 alkane was used as the sole carbon source. In this mutant, a gene was identified upstream of and in the same orientation as almA ( Supplementary Fig. 2a ). This gene encoded a hypothetical protein that displayed 61% identity to a homologue from the SK2 strain and less than 40% homology to sequences from other strains available in GenBank. Following the characterization detailed below, we designated this gene almR , an alkane metabolism regulatory protein gene. To define the function of almR , the MRB5 mutant strain ( almR ) was provided with substrates of various lengths. Disrupting this gene did not significantly affect the growth of the bacterium in the presence of short- or medium-chain alkanes such as C 8 , C 12 , C 16 and C 24 . Inactivation of almR resulted in enhanced growth on LC alkanes, including C 28 , C 32 , C 36 and pristane, compared with the wild-type strain; among the four alkanes, however, the mutation led to more markedly enhanced growth on C 32 ( Supplementary Fig. 3 ). The expression of almR mRNA in the wild-type B5 strain in response to different alkanes was quantified via quantitative PCR. The expression of almR was found to be upregulated relative to the acetate control (showing a 2.4- to 4.8-fold increase) when C 8 , C 12 or C 16 alkanes were used as the sole carbon source. In contrast, induction was not observed when C 24 , C 32 or pristane was used, and almR expression was, in fact, significantly downregulated by C 32 and pristane ( Fig. 2a ). 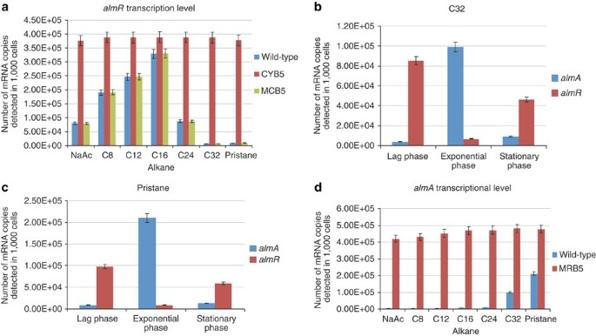Figure 2: Quantification ofalmAandalmRexpression via Q-RT–PCR. The copy number of each mRNA species in 1,000 cells ofA. dieseloleiB5, MRB5 or CYB5 was determined by Q-RT–PCR and normalized to the expression of 16S rRNA. The expression ofalmR(a) andalmA(d) was determined in wild-type B5, CYB5 (cyoD-deficient mutant), MCB5 (mcp-deficient mutant) and MRB5 (almR-deficient mutant) cells. The B5 strain was cultured on the hydrocarbonn-dotriacontane (b) or on pristane (c) and collected during the lag, exponential or stationary growth phase. The data are presented as the mean of three independent experiments. Error bars represent the s.d. Figure 2: Quantification of almA and almR expression via Q-RT–PCR. The copy number of each mRNA species in 1,000 cells of A. dieselolei B5, MRB5 or CYB5 was determined by Q-RT–PCR and normalized to the expression of 16S rRNA. The expression of almR ( a ) and almA ( d ) was determined in wild-type B5, CYB5 ( cyoD -deficient mutant), MCB5 ( mcp -deficient mutant) and MRB5 ( almR -deficient mutant) cells. The B5 strain was cultured on the hydrocarbon n -dotriacontane ( b ) or on pristane ( c ) and collected during the lag, exponential or stationary growth phase. The data are presented as the mean of three independent experiments. Error bars represent the s.d. Full size image The time course of almA and almR expression was monitored from the lag phase to the stationary phase of growth in the wild-type B5 strain growing on pristane or C 32 . The expression of almA was robustly induced by both substrates only during the exponential phase ( Fig. 2b,c ). Conversely, almR expression was significantly inhibited by C 32 and pristane during the exponential phase ( Fig. 2b,c ). Notably, in the MRB5 mutant strain, enhanced almA expression occurred regardless of the presence or absence of alkanes ( Fig. 2d ). CyoD involvement in the modulation of alkane metabolism The CYB5 mutant strain, which is unable to degrade C 32 , exhibits a disrupted copy of CyoD, the subunit of the cytochrome o ubiquinol oxidase (Cyo), which is a putative global transcriptional regulator ( Table 1 ). In the CYB5 mutant strain, the fragment containing the cyoD gene and its flanking regions was sequenced over a length of up to 4.5 kb ( Supplementary Fig. 2b ) and later confirmed via whole-genome sequencing. Growth assays performed in the CYB5 mutant strain in the presence of various alkane substrates demonstrated that interrupting the cyoD gene significantly decreased growth on C 32 , C 36 and pristane and modestly reduced growth on C 28 . In contrast, the CYB5 mutant strain grew more vigorously than the wild-type B5 strain on alkanes with lengths of C 8 –C 24, including C 12 and C 16 ( Supplementary Fig. 3 ). Quantitative reverse transcription–PCR (Q-RT–PCR) revealed that cyoD expression was significantly downregulated (13–18% of that in the acetate control) when the B5 strain was grown using C 8 , C 12 , C 16 or C 24 as the sole carbon source, whereas it was upregulated in the presence of C 28 , C 32 and pristane ( Fig. 3 ). Quantification of the expression data indicated that when cyoD was disrupted in the CYB5 mutant, almR was constitutively expressed at a higher level than in the wild-type B5 strain ( Fig. 2a ). 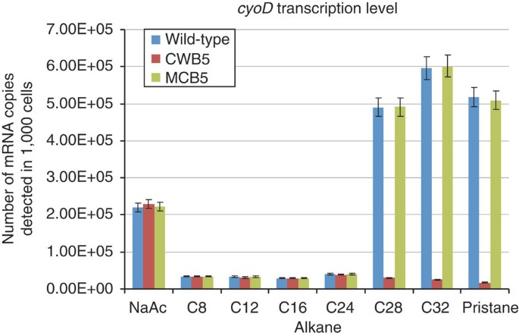Figure 3: Q-RT–PCR analysis ofcyoDexpression in wild-type B5, CWB5 (cheW2-deficient mutant) and MCB5 (mcp-deficient mutant) cells grown on NaAc and other substrates as the sole carbon source. The mRNA expression in 1,000A. dieseloleiB5 cells was determined via Q-RT–PCR and normalized to the expression of the 16S rRNA gene. The data are presented as the mean of three independent experiments. Error bars represent the s.d. Figure 3: Q-RT–PCR analysis of cyoD expression in wild-type B5, CWB5 ( cheW2 -deficient mutant) and MCB5 ( mcp -deficient mutant) cells grown on NaAc and other substrates as the sole carbon source. The mRNA expression in 1,000 A. dieselolei B5 cells was determined via Q-RT–PCR and normalized to the expression of the 16S rRNA gene. The data are presented as the mean of three independent experiments. Error bars represent the s.d. Full size image The roles of mcp , cheR and cheW in alkane utilization In the mutant library, three genes were identified in a chemotaxis operon. These genes encode a methyl-accepting chemotaxis protein (MCP), a methyltransferase (CheR) and a CheW-like signal transduction protein (designated herein as CheW2; Supplementary Fig. 2c ). Interruption of any of these genes significantly reduced bacterial growth in the presence of C 32 . The genes flanking the insertions contained the entire set of chemotaxis proteins within a 13.2-kb region ( Supplementary Table 2 ). This MCP region comprises eight genes encoding cytoplasmic chemotaxis proteins, including MCP, CheW, CheA, CheY1, CheR and CheB. Interestingly, two homologues of CheW and CheY were found in the same region ( Supplementary Fig. 2c and Supplementary Note ). To understand the roles of mcp , cheR and cheW2 in metabolizing alkanes, the growth of deficient strains (MCB5/ mcp , CRB5/ cheR , CWB5/ cheW2 ; Table 1 ) was assayed in the presence of various alkanes. When mcp or cheR was disrupted, growth was decreased significantly in the presence of all of the tested alkanes (C 8 –C 36 and pristine; Supplementary Fig. 5 ). Interestingly, disruption of cheW2 inhibited growth only on LC alkanes longer than C 24 (C 24 –C 36 ) and pristane, whereas normal growth occurred in the presence of alkanes shorter than C 24 (tested with C 8 –C 16 alkanes, Supplementary Fig. 5 ). Expression of chemotaxis genes in response to alkanes The quantitative PCR results revealed that mcp , cheA , cheB , cheR , cheY1 and cheY2 were upregulated in the wild-type B5 strain when grown on C 8 –C 32 n -alkanes or pristane compared with the control (acetate as the sole carbon source; Fig. 4a ). In contrast, cheW1 expression was significantly induced in the B5 strain only in the presence of C 8 –C 24 n -alkanes, whereas cheW2 expression increased significantly in the presence of pristane and n -alkanes longer than C 24 ( Fig. 4a ). Interestingly, when the cyoD gene was interrupted, the levels of mcp , cheA , cheB , cheR , cheY1, cheY2 , cheW1 and cheW2 expression were the same as in the wild-type B5 strain ( Fig. 4a,b ). In addition, when mcp was disrupted, cyoD and almR were expressed at the same level as in the wild-type B5 strain ( Figs 2a and 3 ). However, when the expression of cheW2 was interrupted in the CWB5 mutant strain, no induction of cyoD by LC alkanes (C 28 –C 32 ) and pristane occurred; instead, cyoD expression was significantly repressed ( Fig. 3 ). Conversely, interruption of the cyoD gene had no effect on cheW2 expression ( Fig. 4b ). 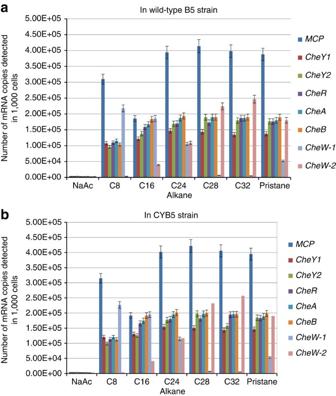Figure 4: The differential expression of chemotaxis genes in response to different alkanes. The expression ofmcp,cheY1,cheY2,cheR,cheA,cheB,chew1andchew2in wild-type B5 (a) and thecyoD-deficient mutant CYB5 (b). The wild-type B5 and the CYB5 strains were grown on different carbon sources; the control cells were cultured on sodium acetate. The data are presented as the mean of three independent experiments. Error bars represent the s.d. Figure 4: The differential expression of chemotaxis genes in response to different alkanes. The expression of mcp , cheY1 , cheY2 , cheR , cheA , cheB , chew1 and chew2 in wild-type B5 ( a ) and the cyoD -deficient mutant CYB5 ( b ). The wild-type B5 and the CYB5 strains were grown on different carbon sources; the control cells were cultured on sodium acetate. The data are presented as the mean of three independent experiments. Error bars represent the s.d. Full size image The roles of mcp , cheR and cheW2 in alkane chemotaxis The alkane chemotaxis behaviour of the wild-type B5 strain and three mutant strains (MCB5/ mcp , CRB5/ cheR , CWB5/ cheW2 ) was evaluated through both capillary and densitometric assays. The quantitative results of these two methods were comparable. The densitometric technique provided quantitative data on the rate of motion on various alkanes. For the wild-type B5 strain, the speed of motion in the presence of different alkanes ranged from 0.43 mm min −1 for C 32 to 0.97 mm min −1 for C 16 ( Fig. 5a ). However, in the MCB5, CRB5 and OMB5 mutant strains, no significant detectable chemotaxis was observed towards any of the tested alkanes. In the CWB5 mutant strain, the recorded speeds were 0.82 and 0.89 mm min −1 in the presence of C 12 and C 16 , respectively, but no significant chemotactic attraction was observed in the presence of C 24 , C 32 or pristane ( Fig. 5a ). Similar results were obtained in the capillary assays ( Fig. 5b ). All three genes contributed to the observed chemotactic behaviour, but cheW2 was specific for LC and branched alkanes. In addition, isothermal titration calorimetry (ITC) was used to evaluate the interaction between MCP and alkanes at 20 °C. The results showed that MCP bound to all of the tested alkanes (C 8 –C 32 alkanes and pristane) but not to acetate ( Table 2 and Supplementary Fig. 6a ). 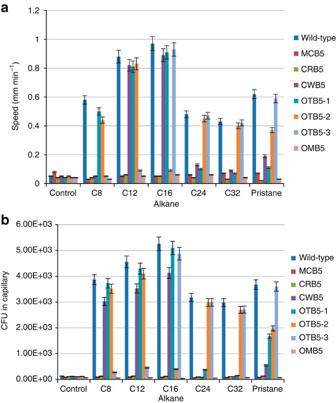Figure 5: The influence of gene mutations on B5 chemotactic behavior towards different alkanes. Chemotaxis of theA. dieseloleiB5 (wild-type) and mutant (MCB5,mcp-deficient mutant; CRB5,cheR-deficient mutant; CWB5,cheW2-deficient mutant; OTB5-1,ompT-1-deficient mutant; OTB5-2,ompT-2-deficient mutant; OTB5-3,ompT-3-deficient mutant and OMB5,ompS-deficient mutant) strains towardsn-alkanes measured via (a) densitometric assays and (b) capillary assays. The data are presented as the mean of three independent experiments. Error bars represent the s.d. Figure 5: The influence of gene mutations on B5 chemotactic behavior towards different alkanes. Chemotaxis of the A. dieselolei B5 (wild-type) and mutant (MCB5, mcp -deficient mutant; CRB5, cheR -deficient mutant; CWB5, cheW2 -deficient mutant; OTB5-1, ompT-1 -deficient mutant; OTB5-2, ompT-2 -deficient mutant; OTB5-3, ompT-3 -deficient mutant and OMB5, ompS -deficient mutant) strains towards n -alkanes measured via ( a ) densitometric assays and ( b ) capillary assays. The data are presented as the mean of three independent experiments. Error bars represent the s.d. Full size image Table 2 In vitro thermodynamic parameters for the binding of different alkanes to OmpS and MCP*. Full size table The expression of three OmpTs A gene encoding an outer membrane transport protein ( orf B5T_02055, designated ompT-1 ) was identified upstream of almR in the same orientation ( Table 1 and Supplementary Fig. 2a ). The transposon mutant screen resulted in the isolation of two additional mutants, ompT-2 ( orf B5T_02580) and ompT-3 ( orf B5T_00277; Table 1 ). All three OmpT proteins were most closely related to putative fatty acid transporters found in Alcanivorax . They showed the highest similarities, 67, 50 and 67%, to the corresponding homologues from Alcanivorax sp. DG881 ( Table 1 ). Q-RT–PCR analysis indicated that ompT-1 expression was strongly upregulated by C 24 –C 32 n -alkanes and pristane in the B5 strain (12.6- to 21.2-fold increase compared with the control), whereas it was only weakly induced by short- and medium-chain n -alkanes (C 8 –C 16 ; 4.2- to 5.9-fold increase compared with the control; Fig. 6a ). However, both ompT-2 and ompT-3 were significantly induced by all the tested alkanes, including the C 8 –C 32 alkanes and pristane (11.7- to 41.9-fold increase compared with the control; Fig. 6a ). 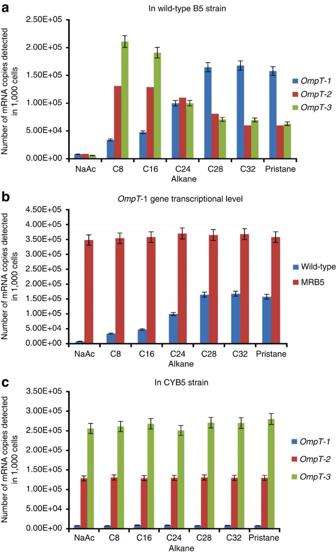Figure 6: The expression ofompT-1,ompT-2andompT-3in theA. dieseloleiB5 (wild-type) and mutant strains grown on various carbon sources and in control cells grown on sodium acetate. The data are presented as the mean of three independent experiments. Error bars represent the s.d. (a) The expression ofompT-1,ompT-2andompT-3in wild-type B5 cells. (b) The expression ofompT-1in wild-type B5 and MRB5 (almR-deficient mutant) cells. (c) The expression ofompT-1,ompT-2andompT-3in CYB5 (cyoD-deficient mutant) cells. Figure 6: The expression of ompT-1 , ompT-2 and ompT-3 in the A. dieselolei B5 (wild-type) and mutant strains grown on various carbon sources and in control cells grown on sodium acetate. The data are presented as the mean of three independent experiments. Error bars represent the s.d. ( a ) The expression of ompT-1 , ompT-2 and ompT-3 in wild-type B5 cells. ( b ) The expression of ompT-1 in wild-type B5 and MRB5 ( almR -deficient mutant) cells. ( c ) The expression of ompT-1 , ompT-2 and ompT-3 in CYB5 ( cyoD -deficient mutant) cells. Full size image Interestingly, disruption of almR increased ompT-1 expression in both the absence and presence of alkanes ( Fig. 6b ), indicating that AlmR downregulates ompT-1 expression. The expression of ompT-2 and ompT-3 in the almR mutant was also analysed, and the interruption of almR did not influence the expression of ompT-2 or ompT-3 ( Supplementary Fig. 7 ). In addition, interruption of the cyoD gene led to the constitutive expression of ompT-2 and ompT-3 in the CYB5 strain in both the absence and presence of alkanes (short or long, straight or branched), suggesting that CyoD downregulates the expression of ompT-2 and ompT-3 ( Fig. 6c ). Selective uptake of alkanes by different OmpTs To determine the roles of various OmpTs in alkane assimilation, the mutant strains OTB5-1, OTB5-2 and OTB5-3, which exhibit disruptions in ompT-1 , ompT-2 and ompT-3 , respectively, were tested for their ability to grow on various n -alkanes (C 8 –C 36 ). The OTB5-1 strain ( ompT -1 mutant) failed to grow on C 28 , C 32 , C 36 or pristane but exhibited nearly normal growth rates on C 8 , C 12 , C 16 and C 24 n -alkanes ( Supplementary Fig. 8 ). In contrast, the OTB5-2 strain did not grow on C 16 or C 24 alkanes but showed weak growth on alkanes with a chain length of <C 16 or >C 24 . Finally, the ompT-3 -interrupted strain (OTB5-3) did not grow on C 8 or C 12 alkanes, grew normally on C 16 and C 24 alkanes and pristane and exhibited a slightly reduced growth rate on C 28 –C 36 alkanes ( Supplementary Fig. 8 ). To verify the function of OmpTs in the selective transport of alkanes, three carbon isotope-labelled alkanes representing short-chain, medium-chain and LC alkanes were utilized in transport assays, as described in the Methods. Based on the measurement of isotopic carbon ( δ 13 C) levels, the amount of isotope-labelled alkane absorbed by the cells was calculated. When the ompT-1 gene was interrupted, the cells transported C 12 and C 16 as efficiently as the wild-type strain ( Fig. 7a,b ) but displayed deficient dotriacontane uptake ( Fig. 7c ). The ompT-2 -knockout cells (strain OTB5-2) could not take up hexadecane ( Fig. 7b ) but transported C 12 and C 32 normally ( Fig. 7a,c ). The ompT-3 gene mutation resulted in an inability of the OTB5-3 strain to transport dodecane ( Fig. 7a ) but had no influence on the uptake of the other two alkanes ( Fig. 7b,c ). 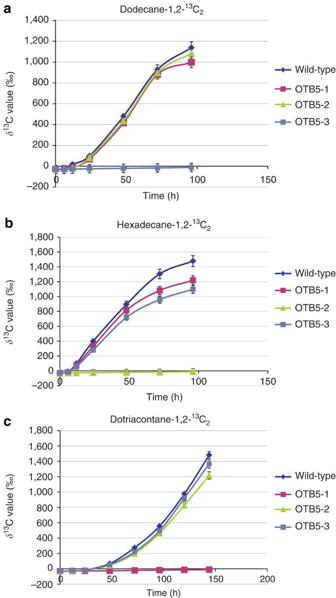Figure 7: Transport assays using isotope-labelledn-alkanes in the wild-type B5 strain and in the OTB5-1 (ompT-1-deficient mutant), OTB5-2 (ompT-2-deficient mutant) and OTB5-3 (ompT-2-deficient mutant) strains. (a) Dodecane-1,2-13C2; (b) hexadecane-1,2-13C2; (c) dotriacontane-1,2-13C2. The data are presented as the mean of three independent experiments. Error bars represent the s.d. Figure 7: Transport assays using isotope-labelled n -alkanes in the wild-type B5 strain and in the OTB5-1 ( ompT-1 -deficient mutant), OTB5-2 ( ompT-2 -deficient mutant) and OTB5-3 ( ompT-2 -deficient mutant) strains. ( a ) Dodecane-1,2- 13 C 2 ; ( b ) hexadecane-1,2- 13 C 2 ; ( c ) dotriacontane-1,2- 13 C 2 . The data are presented as the mean of three independent experiments. Error bars represent the s.d. Full size image OmpT gene interruption abolished chemotaxis to alkanes We suspect that the alkanes bound by MCP within the periplasm are transported by OmpTs across the outer membrane and then trigger chemotaxis. To test this hypothesis, the chemotactic behaviour of the three ompT mutant strains (OTB5-1, OTB5-2 and OTB5-3) were examined in the presence of alkanes with various chain lengths, using both capillary and densitometric assays. The OTB5-1 strain showed no obvious chemotactic attraction to the presence of C 24 , C 32 or pristane because of the interruption of ompT -1 ( Fig. 5 ). In contrast, in the OTB5-2 and OTB5-3 strains, no significant chemotactic attraction was observed in the presence of C 16 or C 12 because of the interruption of ompT -2 or ompT -3, respectively ( Fig. 5 ). The role of OmpS in alkane utilization Another outer membrane protein was found to be essential for alkane utilization. Interruption of this gene led to an inability of the B5 strain to grow on any of the tested alkanes, including C 8 to C 36 and pristane ( Supplementary Fig. 9 ). The identified gene was orf B5T_01485, designated as ompS , and the corresponding mutant strain was denoted as OMB5 ( Table 1 ). OmpS is thought to be a receptor protein because it shares conserved domains (although low overall sequence identity) with a TonB-dependent receptor protein in Escherichia coli that is responsible for ferric citrate transport (EGD69624). In GenBank, this OmpS shows the highest similarity (72%) to a putative outer membrane protein (YP_693408) of A. borkumensis SK2 ( Table 1 ). Gene expression of ompS in the presence of different alkanes was examined to determine its role in alkane assimilation. Unexpectedly, the ompS gene displayed the same transcriptional level as that in the acetate treatment control when the bacterium B5 was exposed to n -alkanes (C 8 –C 36 ) and pristane ( Supplementary Fig. 10a ). Notably, disruption of the ompS gene led to a lack of expression of chemotaxis genes, including mcp , cheA , cheB , cheR , cheY1, cheY2 , cheW1 and cheW2 , in response to all of the tested alkanes ( Supplementary Fig. 10b ). In addition, ompS disruption led to the abnormal expression of other genes, including ompT-1 , ompT-2 , ompT-3 , cyoD , almR , alkB1 , alkB2 and almA , in response to all the tested alkanes ( Supplementary Fig. 10c and d). ITC was also used to determine the interaction between OmpS and alkanes. The results showed that OmpS bound to all the tested alkanes, and the K d values at 20 °C were 7.96±1.42, 6.85±2.05, 5.85±2.21, 6.36±1.74, 7.61±2.30, 8.74±3.49, 11.23±4.66 and 9.71±2.92 μM for the C 8 –C 32 alkanes and pristane, respectively ( Table 2 and Supplementary Fig. 6b ). In the control, OmpS did not bind to acetate ( Supplementary Fig. 6c ). The early responses of bacterial cells to alkane exposure are poorly understood. In this study, key factors involved in alkane sensing, chemotaxis, uptake and regulation, including OmpS, MCP, CheR, CheW, OmpT and AlmR, were identified in the B5 strain. The responses studied herein occur before the onset of hydroxylase-initiated alkane degradation and include alkane sensing, signal transduction and cross-membrane transport. The signal transduction pathways involved are integrated into a network that begins with the alkane stimulus, leading to selective alkane uptake and converging on a specialized degradation pathway for alkanes of different chain lengths. In this study, we found that the outer membrane protein OmpS was essential for alkane degradation. As mentioned above, the OmpS protein of the B5 strain was most closely related to a TonB-dependent receptor protein in E. coli . This protein is responsible for ferric citrate transport across the outer membrane and for initiating a signalling cascade from the cell surface through its outer membrane domains to its N-terminal domain located in the periplasm [37] , [38] . However, our results indicate that OmpS is a signal transmitter and most likely the first sensor of alkanes outside the cell. When ompS was disrupted, the B5 strain failed to grow on all tested alkanes; moreover, there was a lack of expression of all of the genes encoding chemotaxis complex proteins, even in the presence of alkanes. Thus, the mechanism by which OmpS transmits signals to control the expression of chemotaxis genes remains to be further investigated. In strain B5, chemotaxis clearly plays an important role in alkane sensing and subsequent uptake. However, the mechanism underlying alkane chemotaxis is unknown. Before this study, several specific MCP-encoding genes have been found in alkane-degrading bacteria. For example, the tlpS gene, which is situated downstream of alkB1 in the P. aeruginosa PAO1 genome, is predicted to encode the chemotaxis protein MCP [27] . Similarly, an MCP homologue has been identified in P. putida GPo1 (ref. 39 ). Our data confirmed for the first time that the MCP system is indispensable in alkane chemotaxis and also essential for alkane metabolism. Interruption of the mcp gene in strain B5 inhibited growth in the presence of all the tested alkanes, as did the cheR mutation ( Supplementary Fig. 5 ). However, we found that MCP was not essential for alkane signal transduction from the outer membrane to the intracellular regulatory system, as disruption of mcp did not alter cyoD or almR expression in response to LC alkanes ( Figs 2a and 3 ). Instead, CheW appeared to be more critical for signal transduction; in the absence of CheW2, cyoD failed to be expressed ( Fig. 3 ). Intriguingly, the genome of the B5 strain encodes two CheW genes in a single mcp gene cluster. CheW1 was induced by short- and medium-chain alkanes (C 8 –C 24 ), whereas CheW2 was induced only by LC alkanes (C 24 –C 32 ) and pristane ( Fig. 4a ). CheW is essential for chemotactic signal transduction in numerous bacteria, including E. coli , Salmonella typhimurium, Bacillus subtilis, Helicobacter pylori , Myxococcus xanthus and Rhodobacter sphaeroides [40] , [41] , [42] , [43] , [44] , [45] . CheW couples MCP to the histidine kinase CheA [46] . Recently, high-resolution structures of the core signalling complex and the receptor array have been obtained using cryo-electron tomography in E. coli [45] , [47] . In this complex, a CheA/CheW dimer bridges two adjacent receptor trimers (MCP), and three CheA/CheW complexes form a ring that acts as the signalling core. Interestingly, the hexameric rings can be composed solely of CheW [45] . The complex shows a 6:2:1 stoichiometry (six MCP dimers and two CheW monomers for each CheA dimer) [48] . Before this study, little was known about CheW except for its role as a coupling protein. Here, we have determined that CheW plays a critical role in signal transduction from OmpS to Cyo. Interestingly, CheW exhibited differential expression in response to alkanes of varying lengths ( Fig. 4a ), and disruption of cheW2 blocked LC alkane signal transduction to the Cyo terminal oxidase ( Fig. 3 ). In contrast to the differential expression of cheW1 and cheW2 , all the other examined chemotaxis proteins, including mcp , cheA , cheB , cheR , cheY1 and cheY2 , were upregulated in the B5 strain in response to all types of alkanes, including C 8 –C 32 alkanes and pristane ( Fig. 4a ). Moreover, this chemotaxis complex is indispensable for alkane chemotaxis of the B5 strain ( Supplementary Fig. 2 ). Nevertheless, as mentioned above, OmpS may be the first sensor of alkanes, playing an essential role in the expression of chemotaxis proteins. As a generally recognized chemoreceptor, we propose that MCP in the chemotaxis complex is only responsible for sensing alkanes in the periplasm, which are imported by OmpTs, as discussed below. The inactivation of any OmpT leads to insensitivity of the B5 strain to alkanes of specific chain lengths ( Fig. 5 ). To our knowledge, these results are the first evidence supporting the relationship between OmpS, OmpT and MCP in the process of chemotaxis. Previously, we identified three alkane monooxygenases in strain B5. Among them, the two AlkBs engaged in C 12 –C 28 alkane oxidization, and P450 was responsible for C 8 –C 16 n -alkanes [22] . However, the enzyme that mediates LC alkane degradation had not yet been identified. Here we provide evidence that AlmA serves as the hydroxylase for both LC and branched alkanes. The purified enzyme was found to be active and to hydrolyse C 14 –C 36 n -alkanes and pristane, and a high-specific activity was observed on C 24 –C 36 and pristane alkanes ( Fig. 1 and Supplementary Fig. 4 ). However, the LC alkane monooxygenase LadA in Geobacillus thermodenitrificans NG80-2 displayed a high-specific activity only on C 15 –C 28 alkanes and only marginal activity towards C 32 and C 36 alkanes [49] . When almA was disrupted, the B5 strain failed to grow on C 32 –C 36 alkanes ( Supplementary Fig. 3 ), confirming that almA is essential for the degradation of C 32 and longer LC alkanes. The expression of almA was shown to be directly modulated by the negative regulatory protein AlmR ( Fig. 2d ), which does not exhibit homology to any previously described protein. Interestingly, AlmR downregulated the expression of both almA and ompT-1 simultaneously ( Figs 2d and 6b ). This pathway was observed to be specialized for LC and branched alkanes. The occurrence of LC and branched alkanes significantly decreased almR expression and subsequently enhanced the expression of almA and ompT-1 ( Figs 2 and 6 ). In the B5 strain, the Cyo terminal oxidase is situated between the chemotaxis and metabolism pathways and negatively controls the expression of regulator genes associated with different alkane utilization pathways. Based on the annotated genome of the B5 strain, we know that CyoD is the fourth subunit of Cyo. Both the results of previous reports and our work suggest that Cyo participates in the regulation of alkane-degradation pathways. However, the exact underlying mechanism remains unknown. According to investigations with P. putida , the expression of Cyo genes is influenced by the level of oxygen as well as the catabolic repression of simple carbon sources such as succinate and lactate [50] , [51] . Inactivation of cyo affects the expression of the genes encoding organic acid transporters, porins, transcriptional regulators, terminal oxidases and many others [34] . However, the process by which the activity of Cyo is transformed into a transcriptional regulation signal remains unknown [13] . In this report, we found that cyo was differentially expressed in response to different carbon sources ( Fig. 3 ). The most intriguing phenomenon was the contrast in cyo expression in response to alkanes of different chain lengths. In strain B5, Cyo was only partially repressed by acetate as the simple carbon source, exhibiting approximately half of the expression level compared with expression in the presence of LC alkanes (C 28 , C 32 ) and pristane. However, in the presence of short- to medium-chain lengths (C 8 –C 24 ), the expression level of Cyo was almost completely repressed to levels equivalent to the alkane chemotaxis null mutant lacking chew2 , potentially representing background expression ( Fig. 3 ). We also confirmed that Cyo is essential for relaying the signal from CheW to the alkane degradation pathways. Cyo downregulated the expression of the negative regulator AlmR ( Fig. 2a ), and interruption of cyoD resulted in the constitutive expression of ompT-2 and ompT-3 ( Fig. 6 ). Phenotypically, disruption of cyoD significantly decreased growth of the B5 strain on C 28 –C 36 alkanes and on pristane but increased growth on C 8 –C 24 alkanes compared with the wild-type B5 strain ( Supplementary Fig. 3 ). Taken together, these results suggest that Cyo is involved in the modulation of alkane utilization. Before this study, although proteins that allow the passage of aromatic hydrocarbons across the outer membrane had been identified [33] , [34] , [35] , [36] , there was little compelling evidence for the transport of aliphatic hydrocarbons across the cytoplasmic membrane. In the B5 strain, three OmpTs were confirmed to be responsible for alkane transport ( Fig. 7 ). OmpT is reported to encode a putative LC fatty acid transporter that belongs to the FadL family, members of which are common in Gram-negative bacteria capable of xenobiotic biodegradation [33] . The other two proteins are the xylene transporter (XylN) of P. putida and the toluene transporter (TbuX) of Ralstonia pickettii PK01, which also belong to the FadL family [35] , [36] . Our results indicate that different OmpTs can selectively transport different alkanes. OmpT-1 would be responsible for the uptake of C 28 –C 36 n -alkanes, OmpT-2 for medium-chain (C 16 –C 24 ) n -alkanes and OmpT-3 for C 8 –C 12 n -alkanes ( Fig. 7 ). When alkanes were present, specific ompT gene expression was activated via the signal transduction system as discussed above ( Fig. 6 ) to allow the transport of the corresponding alkanes across the outer membrane ( Fig. 7 ). However, when a simple carbon substrate such as acetate was present, the expression of all the ompT genes was significantly decreased ( Fig. 6a ). In summary, we gained novel insight into the mechanisms associated with alkane degradation in Alcanivorax dieselolei . Several key factors involved in alkane sensing and uptake were identified in this report, in addition to the LC alkane hydroxylase, AlmA, and the regulator AlmR. A signal transduction network is proposed based on factors involved in alkane sensing, uptake and oxidization and in the regulation of gene expression. This network extends from an outer membrane receptor protein to the chemotaxis system, then to the global regulation of gene expression and, finally, to the regulation of LC alkane degradation. As illustrated schematically ( Fig. 8 ), the first step in this proposed pathway is the sensing of alkanes outside of the cell by OmpS, which triggers the expression of chemotaxis complex protein genes that are specialized for alkanes. Subsequently, CheW delivers the alkane stimulus to the global regulation system and induces Cyo expression via a mechanism that remains to be unraveled. In the case of LC alkanes, the elevated expression of Cyo represses almR expression, thereby counteracting the negative effects of AlmR. In turn, OmpT-1 expression is induced, initiating the transport of LC alkanes across the outer plasma membrane. The accumulated alkanes in the periplasm contact MCP and initiate chemotaxis. Meanwhile, the expression of almA is initiated, resulting in the oxidation of LC alkanes. Corresponding pathways also exist for short- and medium-chain alkanes and involve CheW1, OmpT2/3 and specific regulators (not included in Fig. 8 ). Further studies using transcriptomic or proteomic approaches will confirm and refine our understanding of the connections between alkane sensing and gene expression regulation that are likely bridged by CheW. 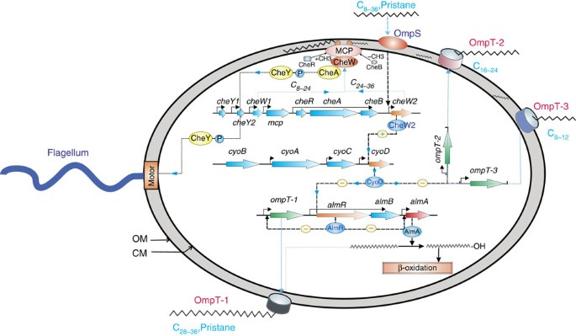Figure 8: Proposed regulation of LC-alkane metabolism inA. dieseloleiB5. The predicted sensing proteins and chemotactic pathways for alkanes are charted at the top of the diagram. The predicted regulatory pathways for LC alkane degradation are charted in the middle of the diagram. The LC alkane utilization pathways are charted at the bottom of the diagram. The predictedn-alkane transporters are labelled in the lower left and upper right corners of the diagram. The known functional pathways are represented as solid lines. The unknown or uncertain functional pathways are represented by dashed lines. The plus sign surrounded by a circle represents positive regulation. The minus sign surrounded by a circle represents negative regulation. OM, outer membrane; CM, cytoplasm membrane (inner membrane). Figure 8: Proposed regulation of LC-alkane metabolism in A. dieselolei B5. The predicted sensing proteins and chemotactic pathways for alkanes are charted at the top of the diagram. The predicted regulatory pathways for LC alkane degradation are charted in the middle of the diagram. The LC alkane utilization pathways are charted at the bottom of the diagram. The predicted n -alkane transporters are labelled in the lower left and upper right corners of the diagram. The known functional pathways are represented as solid lines. The unknown or uncertain functional pathways are represented by dashed lines. The plus sign surrounded by a circle represents positive regulation. The minus sign surrounded by a circle represents negative regulation. OM, outer membrane; CM, cytoplasm membrane (inner membrane). Full size image Bacterial strains and primers The bacterial strains, plasmids and oligonucleotide primers utilized in this study are listed in Supplementary Table 3 and the Supplementary Methods . The nucleotide sequence of the complete A. dieselolei B5 genome has been previously reported and is available in GenBank (accession code CP003466 ) [29] . Construction of a mini-Tn5 transposon library The method applied for transposon mutagenesis was based on the mini-Tn5 Str/Sp element, which was constructed as previously described [52] . The A. dieselolei B5 strain was grown in modified Luria-Bertani (LB) medium until the stationary growth phase, and the cells were then centrifuged at 3,200 g at 4 °C. The E. coli donor (CC118 λ pir) and helper (HB101) strains were grown overnight at 37 °C in LB medium containing streptomycin, washed with fresh LB and centrifuged at 3,200 g at 4 °C. The pellets obtained from the A. dieselolei B5 strain and the E. coli donor and helper strains were mixed at a 4:1:1 ratio (by volume) and placed on a membrane filter on a plate containing LB agar, salts (0.45 gl −1 Na 2 HPO 4 ·2H 2 O, 2.5 gl −1 NaNO 3 , 11.5 gl −1 NaCl, 0.38 gl −1 KCl and 0.7 gl −1 CaCl 2 ·2H 2 O) and 2% (wt/vol) acetate as a carbon and energy source. The plates were incubated for 24 h at 30 °C, and the cells were then washed with 10 mM MgSO 4 . Finally, transconjugants were selected on modified LB medium containing 0.5% (wt/vol) acetate as a carbon source with nalidixic acid (0.01 mg ml −1 ) and streptomycin as required. A transposon library consisting of approximately 20,000 colonies was obtained based on the mini-Tn5 transposon element. The A. dieselolei B5 genome contains 4,448 genes [29] . This library therefore displayed approximately fivefold coverage of the genome. However, mutant clones with identical disrupted genes were isolated, indicating that the library was most likely saturated. The quality of the library was verified by Southern blot hybridization, which confirmed the randomness and uniqueness of the transposon insertions. High-throughput screening of mutant library Transposon mutants from the 96-well library plates were replicated in OmniTray plates (Nunc) containing solid artificial sea water medium (ASM) without a carbon source (24 g NaCl, 7.0 g MgSO 4 ˙7H 2 O, 1 g NH 4 NO 3 , 0.7 g KCl, 2.0 g KH 2 PO 4 , 3.0 g Na 2 HPO 4 and 10 ml of a trace element solution, pH 7.5). Following transfer of the mutants, a C 32 alkane powder was added to the OmniTray plates as previously described [11] . The plates were incubated at 30 °C for 48 h, and growth was detected by overlaying the plates with top agar containing 0.05% (wt/vol) iodonitrotetrazolium chloride. The reduction of iodonitrotetrazolium chloride by the active respiratory chain of growing cells resulted in purple staining of the colonies [53] . Mutants exhibiting no growth or abnormal growth on C 32 alkane were re-arrayed from the original library into new 96-well microtitre plates containing 200 μl of modified LB medium supplemented with nalidixic acid and streptomycin. The plates were incubated overnight at 30 °C at 900 r.p.m. The resulting library was enriched for mutants that either showed an abnormal ability to utilize C 32 or were unable to use C 32 as a carbon source. To confirm the results of the initial screening and further analyse these mutants, they were replicated in OmniTray plates containing ASM supplemented with 0.5% (wt/vol) sodium acetate or with C 16 or C 32 alkanes as the sole carbon source. Mutants exhibiting no growth or abnormal growth on C 32 but wild-type growth on plates supplemented with acetate were chosen for further analysis. Growth experiments To test the growth of the mutants on various alkane substrates, the wild-type B5 and mutant strains were grown in 100 ml of ASM containing the appropriate antibiotics in 250 ml Erlenmeyer flasks at 28 °C on a rotary shaker (200 r.p.m.). Alkanes were added in the form of either 350 μl of liquid alkanes (C 8 , C 12 , C 16 and pristane) or 0.1% (w/v) solid alkane (C 18 , C 24 , C 28 , C 32 and C 36 ) per 100 ml of ASM medium. Detailed procedures are provided in the Supplementary Methods . Inverse PCR and real-time PCR The mini-Tn5 insertion sites in the selected mini-Tn5 mutants were identified via inverse PCR. To evaluate gene expression, the number of mRNA copies present in 1,000 A. dieselolei B-5 or mutant cells was determined using quantitative real-time PCR. The details of these procedures are described in the Supplementary Methods . Chemotaxis assays Preparation of chemoeffector solutions . Alkane solutions were prepared by saturating the chemotaxis buffer (410.75 mM NaCl, 9.39 mM KCl, 21.5 mM Na 2 HPO 4 , 22.41 mM KH 2 PO 4 and 0.123 mM EDTA, pH 7.0 ) with excess crystals for several days and then passing them through polycarbonate filters (0.45 μm) to remove the remaining solid alkanes (maintained at 10 °C). The aqueous solubilities of the tested alkanes are as follows (mol l −1 ) [54] : 5 × 10 −7 for nonane, 2 × 10 −8 for dodecane, 2 × 10 −10 for hexadecane, 6 × 10 −13 for tetracosane, 4 × 10 −16 for dotriacontane and 3 × 10 −11 for pristane. Densitometric chemotaxis assay . Densitometric chemotaxis assays were performed as previously described [55] with minor modifications. The bacterial strains were cultivated in 50-ml screw-cap tubes containing 20 ml of ASM medium and 0.5% (wt/vol) NaAc as a growth substrate and were maintained at 25 °C on a rotary shaker (180 r.p.m.). Microbial cultures from the mid-exponential growth phase were centrifuged at 5,000 g for 10 min, washed three times with potassium phosphate buffer (pH 7.0) and resuspended in the same buffer solution at a final concentration of 10 9 cells ml −1 (OD 600 =0.3). These suspensions were stored at 4 °C for no more than 24 h before the chemotaxis assays were performed. Each densitometric chamber (a 5-ml quartz cuvette) was completely filled with chemotactic buffer solution. An aliquot of the bacterial suspensions (200 μl) was then added to the bottom of the chamber using a micropipette. The control chambers contained only chemotactic buffer solution. The distribution of bacterial cells in the densitometric chamber was monitored at 25 °C at various time intervals using a densitometer (2222-010 Ultrascan XL, LKB Produkter AB). Based on the obtained densitograms, the speed ( V ) of the bacterial front was calculated using the following formula: V =( X n − X 1 )/( t n − t 1 )[mmh −1 ], where X n and X 1 are the positions of the bacterial front at times t n and t 1 , respectively. The experiments were repeated at least three times. Capillary chemotaxis assay . For these assays, the density of the bacterial suspensions, which were prepared as described for the densitometry assays, was brought to approximately 5 × 10 7 cells ml −1 . Following the classical capillary method [55] , these assays were performed by placing a few drops of a suspension in a small chamber consisting of a U-shaped glass tube between a microscope and a coverslip. The chemotactic response was measured by placing the open end of a 1-μl capillary tube containing the chemoeffector solution in the pool of bacterial cells in the chamber. After 30 min of incubation at 30 °C, the contents of the capillaries were transferred to tubes containing ASM medium. The appropriate dilutions were prepared, and 0.1-ml samples were spread on Alcanivorax agar plates. The number of colonies was counted after incubation of the plates at 30 °C for 16–24 h. The presented results are based on the average count obtained from triplicate plates in each of three separate capillary assays and are expressed as the number of cells per capillary. In all experiments, a blank control (without chemoeffector) was included. The relative error in the capillary assays was less than 10%. Cross-membrane transport assays Transport assays involving isotope-labelled n -alkanes were performed using a modified form of the method described by Kumar and Black [56] . The wild-type B5 strain and the OTB5-1, OTB5-2 and OTB5-3 mutant strains were grown in 100 ml of ASM liquid medium containing the appropriate antibiotics. Sodium acetate was used as the sole carbon source, and the strains were maintained in 250-ml Erlenmeyer flasks at 28 °C on a rotary shaker (200 r.p.m.). When the cultures reached OD 600 =0.5, the cells were collected, washed with ASM, resuspended in ASM and starved for 3–5 h at 28 °C. After starvation, the cells were cultured in 100 ml of ASM containing the appropriate antibiotics and dodecane-1,2- 13 C 2 , hexadecane-1,2- 13 C 2 and dotriacontane-1,2- 13 C 2 (Sigma-Aldrich) as the sole carbon sources. The cells were maintained in 250-ml Erlenmeyer flasks at 28 °C on a rotary shaker (200 r.p.m.). When the cultures reached OD 600 =0.5, the cells were collected at the beginning of the experiment (0 h), at intermediate time points (6, 12, 24, 48 and 72 h for dodecane-1,2- 13 C 2 and hexadecane-1,2- 13 C 2 ; 12, 24, 48, 72, 96 and 120 h for dotriacontane-1,2- 13 C 2 ) and at the end of the experiment (96 h for dodecane-1,2- 13 C 2 and hexadecane-1,2- 13 C 2 ; 144 h for dotriacontane-1,2- 13 C 2 ). The cells were then washed three times with fresh ASM medium to remove the residual n -alkane- 13 C 2 , air-dried and subjected to carbon ( δ 13 C) isotopic analysis. Carbon ( δ 13 C) isotopic analyses were performed using a Carlo Erba 1108 Elemental Analyzer (EA) connected via a Conflo II interface to a Finnigan MAT Delta Plus XL isotope ratio mass spectrometer [56] . The EA was operated at an oxidation furnace temperature of 1,020 °C, a reduction furnace temperature of 650 °C and a packed-column temperature of 60 °C. The resulting carbon isotopic values are typically expressed as δ -values (the difference compared with an international standard in parts per thousand) defined as δ 13 C (‰)=( R smpl/ R std−1) × 1,000. R smpl is the 13 C/ 12 C ratio of the sample material, and R std is the 13 C/ 12 C ratio of an International Atomic Energy Authority standard (Vienna Pee Dee Belemnite, for which the 13 C/ 12 C ratio has been defined as the official zero point of the carbon isotopic scale). The carbon ( δ 13 C) isotopic values are presented as ‰ versus the stated standard. Construction of plasmids The plasmid pET- almA (pEA-B5) was constructed by amplifying almA with the B5 almAwf/B5almAwr primer pair ( Supplementary Table 3 ) and cloning the resulting PCR products into the Bam HI/ Hin dIII sites of pET-28a (+) (Novagen). The following PCR programme was utilized for these assays: 95 °C for 3 min, followed by 30 cycles of 95 °C for 30 s, 50 °C for 45 s and 72 °C for 2 min, with a final extension at 72 °C for 5 min. For in vitro experiments, pET- almA was transfected into E. coli BL21 cells (Novagen), and almA was overexpressed and purified as described below. The DNA fragments of the mcp and ompS genes encoding the MCP and OmpS peptides were amplified with primers containing restriction sites for Hin dIII/ Eco RI and Bam HI/ Sac I, respectively ( Supplementary Table 3 ). The following PCR programme was utilized for these assays: 95 °C for 3 min, followed by 30 cycles of 95 °C for 30 s, 50–52 °C for 45 s and 72 °C for 2 min, with a final extension at 72 °C for 5 min. The resulting PCR products were then cloned into pET28a (+). Expression and purification E. coli BL21 cells expressing pET- almA were grown in LB supplemented with 50 mg ml −1 kanamycin at 37 °C with shaking at 150 r.p.m. to approximately A 600 =0.5. The expression of almA was induced by the addition of 0.2 mM isopropyl-β- D -thiogalactoside, followed by incubation for 3 h at 37 °C. The cells were collected via centrifugation at 10,000 g at 4 °C for 3 min and then washed with and resuspended in 50 mM Tris-HCl buffer (pH 7.5). After the addition of phenylmethylsulphonyl fluoride and lysozyme (final concentrations of 1 mM and 1 mg ml −1 , respectively), the cell suspension was incubated for 20 min at 4 °C and then sonicated. Following RNase (10 mg ml −1 ) and DNase (5 mg ml −1 ) treatment for 15 min on ice, cell extracts were obtained via centrifugation at 23,000 g for 20 min at 4 °C. Protein purification was performed using a Ni 2+ -Chelating Sepharose Fast Flow column (Amersham Biosciences) according to the procedure recommended by the manufacturer (QIAGEN). E. coli BL21 (DE3) containing pET28- mcp and pET28- ompS were grown at 37 °C until the culture reached an OD 600 of 0.6. Isopropyl β- D -1-thiogalactopyranoside (0.4 mM) was then added, and the culture was maintained at 30 °C for 3 h. Cellular lysates of recombinant E. coli were prepared by sonification of cell suspensions in 50 mM phosphate buffer (pH 8.0). The proteins were purified using His-affinity resin chromatography according to the manufacturer’s (Novagen) instructions and then further purified by fast protein liquid chromatography on Superdex 200 (Pharmacia). Enzyme assay Purified AlmA was assayed for alkane monooxygenase activity according to the methods described by Maeng et al . with slight modifications [57] . The reaction mixtures contained 50 mM Tris-HCl (pH 7.5), 1 mM hexadecane (or other n -alkanes as indicated), 1 mM each of NADH and MgSO 4 and 10 mg of purified AlmA. The control mixture contained no enzyme. The mixtures were incubated at 60–75 °C with shaking for 5 min before cyclohexane extraction, and the alkane residues in the extract were analysed via GC as previously described [58] . The reaction products were identified through GC–MS (Finnigan Polaris Q; Thermo Fisher Scientific, Inc.) using a DB-5 MS column (30 m × 0.25 mm i.d. and 1 mm thickness; Agilent Technologies). Separation was performed at 120 °C for 1 min, and the temperature was then increased from 120 °C to 280 °C at a rate of 15 °C min −1 . The resultant spectra were recorded in electron impact mode at 70 eV. The specific activity is expressed as U mg −1 of enzyme. One unit was defined as the amount of enzyme required to hydroxylate 1 μmol of alkane per min. Isothermal titration calorimetry ITC was performed as previously described [59] with minimal modifications. Measurements were performed using a NANO ITC 2G at 20 °C. The MCP protein was dialysed against buffer containing 5 mM Tris, 5 mM MES, 5 mM PIPES, 5 mM NaCl and 5 mM imidazole, pH 8.0. The OmpS protein was dialysed against buffer containing 7 mM Tris, 5 mM MES, 3.5 mM PIPES, 6.5 mM NaCl and 5 mM imidazole, pH 7.5. For the ligand-binding analysis, the protein was introduced into the sample cell and titrated with aliquots of ligand solution. For solid alkanes (C 24 , C 28 , C 32 and C 36 ), the ligand solutions were dissolved in hexane. For the OmpS protein ligand-binding analysis, an injection series (2 μl for the first injection and 8 μl for subsequent injections) was conducted using a 250-μl syringe filled with the test solutions (20 injections at 100-min intervals). For the MCP protein ligand-binding analysis, an injection series (2 μl for the first injection and 10 μl for subsequent injections) was conducted using a 250-μl syringe filled with the test solutions (25 injections at 120-min intervals or 16 injections at 100-min intervals). Data were analysed using the NanoAnalyze software package with Independent Model. Because the ITC experiments were conducted in only a single buffer, the binding constants determined may be buffer dependent. How to cite this article: Wang, W. et al . The long-chain alkane metabolism network of Alcanivorax dieselolei . Nat. Commun. 5:5755 doi: 10.1038/ncomms6755 (2014).